DIP1 modulates stem cell homeostasis inDrosophilathrough regulation ofsisR-1 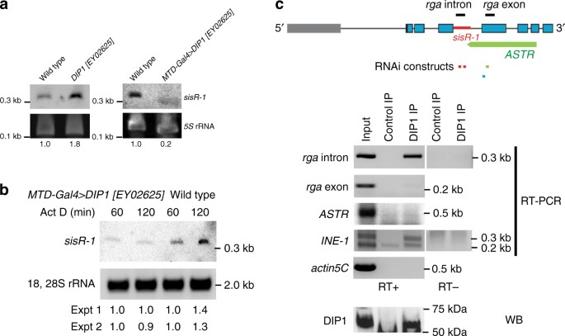Fig. 1 DIP1 regulatessisR-1.aRepresentative northern blots (out of at least three biological replicates) showing the expression ofsisR-1in the ovaries of the indicated genotypes. 5S rRNA was used as a loading control. Numbers below indicate relative band intensities ofsisR-1normalized to rRNA quantified using ImageJ software.bNorthern blot showing the levels ofsisR-1in the ovaries of the indicated genotypes after 60 and 120 min of actinomycin D treatment. 18, 28S rRNA was used as a loading control. Numbers below indicate relative band intensities (120 min compared to 60 min) ofsisR-1normalized to rRNA quantified using ImageJ software from two independent experiments.cRT-PCR and western blot showing enrichment ofsisR-1and INE-1 but notrgaexonic sequences andASTRin DIP1 immunoprecipitated samples.Actin5Cwas used as a negative control for unspecific pull down. The regions where the intronic and exonic sequences were amplified by PCR were shown on thergagene model. Thered linein the intron is wheresisR-1is encoded. Locations of RNAi constructs used to targetsisR-1(red),ASTR(green), andrga(blue) were indicated. WB, western blot Stable intronic sequence RNAs (sisRNAs) are by-products of splicing and regulate gene expression. How sisRNAs are regulated is unclear. Here we report that a double-stranded RNA binding protein, Disco-interacting protein 1 (DIP1) regulates sisRNAs in Drosophila . DIP1 negatively regulates the abundance of sisR-1 and INE-1 sisRNAs. Fine-tuning of sisR-1 by DIP1 is important to maintain female germline stem cell homeostasis by modulating germline stem cell differentiation and niche adhesion. Drosophila DIP1 localizes to a nuclear body (satellite body) and associates with the fourth chromosome, which contains a very high density of INE-1 transposable element sequences that are processed into sisRNAs. DIP1 presumably acts outside the satellite bodies to regulate sisR-1 , which is not on the fourth chromosome. Thus, our study identifies DIP1 as a sisRNA regulatory protein that controls germline stem cell self-renewal in Drosophila . Recent studies have uncovered a class of stable intronic sequence RNAs (sisRNAs) that are derived from the introns post splicing [1] . sisRNAs are present in various organisms such as viruses, yeast, Drosophila , Xenopus , and mammals [1] , [2] , [3] , [4] , [5] , [6] , [7] , [8] , [9] , [10] , [11] . Studies in Drosophila and mammalian cells suggest that sisRNAs function in regulating the expression of their parental genes (host genes where they are derived from) via positive or negative feedback loops [5] , [10] , [11] . In yeast, sisRNAs are involved in promoting robustness in response to stress [7] , while in Drosophila , sisRNAs have been shown to be important for embryonic development [12] . However, very little is understood about the biological functions of sisRNAs in terms of regulating cellular processes such as differentiation, proliferation, and cell death. The Drosophila genome encodes for several double-stranded RNA (dsRNA) binding proteins that localize to the nucleus [13] , [14] . Most of them have been found to regulate specific RNA-mediated processes such as RNA editing, X chromosome activation, and miRNA biogenesis [15] , [16] , [17] , [18] , [19] , [20] . The Disco-interacting protein 1 (DIP1) is a relatively less characterized dsRNA binding protein that has been implicated in anti-viral defense and localizes to the nucleus as speckles. Otherwise, not much is known about the biological processes regulated by DIP1 [21] , [22] , [23] , [24] . In this paper, we show that the regulation of a Drosophila sisRNA sisR-1 by DIP1 is important for keeping female germline stem cell homeostasis in place. We also show that DIP1 regulates INE-1 sisRNAs and localizes to a previously undescribed nuclear body around the fourth chromosomes, called the satellite body. The regulation of sisR-1 , which is not on the fourth chromosome, by DIP1 presumably does not occur in the satellite bodies. DIP1 regulates sisR-1 We previously identified a sisRNA sisR-1 in Drosophila [5] . To identify proteins that regulate sisR-1 abundance, we employed a candidate approach of dsRNA binding proteins that localize to the nucleus [13] . We began by searching for candidate genes that are specific to the sisRNA pathway. In Drosophila , there are seven dsRNA binding proteins that localize to the nucleus [13] . Over the years, many of the original dsRNA binding proteins have been assigned functions to the miRNA and RNAi pathways. For example, CG188 (now pasha ) and drosha , and CG12493 (now blanks ) have been assigned to the miRNA and siRNA pathways respectively [25] , [26] . 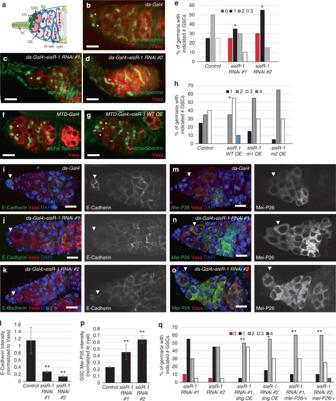Fig. 2 sisR-1regulates GSC–niche occupancy by maintaining GSC–niche adhesion and suppressing GSC differentiation.aA drawing of a germarium. GSC, germline stem cell, CC, cap cell, TF, terminal filament, EC, escort cell, CB, cystoblast.b–d,f–gConfocal images of germaria of the indicated genotypes stained for alpha-Spectrin (green) and Vasa (red).Scale bar: 10 µM.Asterisks(*) mark the GSCs.e,h,qCharts showing the percentages of germaria with the indicated number of GSCs of the indicated genotypes. *P< 0.05, **P< 0.01. Fisher’s exact test.N= 20.i–kConfocal images of germaria of the indicated genotypes stained for E-Cadherin (green), Vasa (red), and DAPI (blue).Arrowheadspoint to GSC–niche interfaces.m–oConfocal images of germaria of the indicated genotypes stained for Mei-P26 (green), Vasa (red), and DAPI (blue).Scale bar, 10 µM.Arrowheadspoint to GSCs.l,pCharts showing the quantification of E-Cadherin and Mei-P26 intensities. **P< 0.01.N= 3.Error barsrepresent s.d. CG12598 (now adar ) and mle have been shown to be required for RNA editing and X-activation respectively [20] , [27] . Among the seven, DIP1 and CG8273 are the least characterized and therefore most promising. The role of CG8273 in sisR-1 regulation will be reported in a separate study. We found that DIP1 functions to reduce the levels of sisR-1 . DIP1 is a dsRNA binding protein that localizes to nuclear speckles and regulates cell fate decisions during development [23] . In DIP1 mutant ovaries, sisR-1 level was upregulated (Fig. 1a and Supplementary Fig. 1a ), suggesting that DIP1 negatively regulates sisR-1 . Since the rga mRNA was downregulated in DIP1 mutant ovaries (Supplementary Fig. 1b ), the upregulation of sisR-1 was not due to increase in rga transcription. Conversely, germline overexpression of DIP1 using a transgenic fly containing an EP element upstream of the 5ʹUTR of the DIP1 locus resulted in a decrease in the abundance of sisR-1 (Fig. 1a and Supplementary Fig. 1a ). These results indicated that DIP1 represses sisR-1 abundance. However, we were not able to perform in situ hybridization to detect sisR-1 in the ovaries due to its low abundance and inability to distinguish sisR-1 from rga pre-mRNA. Fig. 1 DIP1 regulates sisR-1 . a Representative northern blots (out of at least three biological replicates) showing the expression of sisR-1 in the ovaries of the indicated genotypes. 5S rRNA was used as a loading control. Numbers below indicate relative band intensities of sisR-1 normalized to rRNA quantified using ImageJ software. b Northern blot showing the levels of sisR-1 in the ovaries of the indicated genotypes after 60 and 120 min of actinomycin D treatment. 18, 28S rRNA was used as a loading control. Numbers below indicate relative band intensities (120 min compared to 60 min) of sisR-1 normalized to rRNA quantified using ImageJ software from two independent experiments. c RT-PCR and western blot showing enrichment of sisR-1 and INE-1 but not rga exonic sequences and ASTR in DIP1 immunoprecipitated samples. Actin5C was used as a negative control for unspecific pull down. The regions where the intronic and exonic sequences were amplified by PCR were shown on the rga gene model. The red line in the intron is where sisR-1 is encoded. Locations of RNAi constructs used to target sisR-1 ( red ), ASTR ( green ), and rga ( blue ) were indicated. WB, western blot Full size image We next examined whether DIP1 affects the expression of sisR-1 via a transcriptional or post-transcriptional manner. We treated wild-type and DIP1 overexpression ovaries with actinomycin D to inhibit transcription and observed any changes in sisR-1 abundance. Previous analysis showed that a 30 min treatment was sufficient to inhibit transcription in the ovaries [5] . In control ovaries, we observed a strong accumulation of sisR-1 over time from 60 to 120 min post treatment (Fig. 1b ), indicating that mature and stable sisR-1 was being produced from the precursors during this period of time. However, in ovaries overexpressing DIP1 , the accumulation of sisR-1 was perturbed (Fig. 1b ). No observable change was seen for 18, 28S rRNA (Fig. 1b ). This observation suggests that DIP1 may regulate the stability and/or processing of sisR-1 in a post-transcriptional manner. It is interesting to note that a previous study had shown that actinomycin D can inhibit the turnover of a nuclear form of hsr-omega ncRNA in Drosophila [28] . Together with our observation, it implies that actinomycin D may regulate the decay of specific ncRNAs in the nucleus by a yet unknown mechanism. To ask whether the effect of DIP1 on sisR-1 is direct, we checked whether DIP1 interacts with sisR-1 in a complex by performing in vivo co-immunoprecipitation. We generated an antibody against DIP1 (Supplementary Fig. 1c ) and immunoprecipitated endogenous DIP1 in S2 cells (Fig. 1c ). RT-PCR revealed that DIP1 interacted with sisR-1 , but not with the exonic sequences of rga and actin5C as negative controls (Fig. 1c ), suggesting that DIP1 directly regulates the stability of sisR-1 . Moreover, DIP1 did not interact with ASTR , a target of sisR-1 , suggesting that DIP1 is not part of the sisR-1 silencing complex (Fig. 1c ). Thus, DIP1 binds to sisR-1 and regulates steady-state sisR-1 levels in Drosophila . sisR-1 promotes GSC–niche occupancy In Drosophila, sisR-1 had been shown to regulate the expression of its host gene regena ( rga ) [5] . The rga gene had been identified as a candidate gene that regulates germline stem cell (GSC) differentiation in the ovaries [29] . To assess the biological significance of DIP1-mediated regulation of sisR-1 , we therefore examined if sisR-1 regulates GSC self-renewal or differentiation. In the Drosophila germarium, GSCs can be identified by their location in the niche (anterior tip) and the stereotypic location of spherical spectromes at the GSC–niche interface (hereafter referred as GSC–niche occupancy, which means GSCs that are in physical contact with the niche, Fig. 2a, b ). We found that manipulating the expression of sisR-1 using previously reported RNAi lines, which specifically knocked down sisR-1 but not its parental rga gene, changed the GSC–niche occupancy [5] (see “Methods”). Immunostaining showed a decrease in the number of GSCs in two independent sisR-1 RNAi flies compared to controls at day 7 after eclosure (appearance of germaria with 0 GSCs not found in controls, Fig. 2b–e ), suggesting that sisR-1 is required for the maintenance of GSCs in the niche. Fig. 2 s isR-1 regulates GSC–niche occupancy by maintaining GSC–niche adhesion and suppressing GSC differentiation. a A drawing of a germarium. GSC, germline stem cell, CC, cap cell, TF, terminal filament, EC, escort cell, CB, cystoblast. b – d , f – g Confocal images of germaria of the indicated genotypes stained for alpha-Spectrin ( green ) and Vasa ( red ). Scale bar : 10 µM. Asterisks (*) mark the GSCs. e , h , q Charts showing the percentages of germaria with the indicated number of GSCs of the indicated genotypes. * P < 0.05, ** P < 0.01. Fisher’s exact test. N = 20. i – k Confocal images of germaria of the indicated genotypes stained for E-Cadherin ( green ), Vasa ( red ), and DAPI ( blue ). Arrowheads point to GSC–niche interfaces. m – o Confocal images of germaria of the indicated genotypes stained for Mei-P26 ( green ), Vasa ( red ), and DAPI ( blue ). Scale bar , 10 µM. Arrowheads point to GSCs. l , p Charts showing the quantification of E-Cadherin and Mei-P26 intensities. ** P < 0.01. N = 3. Error bars represent s.d. Full size image Previously, sisR-1 was shown to repress the expression of ASTR , possibly via its 3ʹ tail (Supplementary Fig. 2a ) [5] . To test if the 3ʹ end of sisR-1 is required for silencing of ASTR in vivo, we overexpressed wild-type and mutant forms of sisR-1 , and assayed for their ability to repress ASTR . Both m1 and m2 versions of sisR-1 were mutations introduced at different regions of the 3ʹ tail to disrupt complementary base pairing to ASTR (Supplementary Fig. 2b ). Transgene expression was verified by measuring dsRed expression (Supplementary Fig. 2c ). We observed that MTD-Gal4 -induced overexpression of wild-type sisR-1 was indeed more effective than m1 and m2 in repressing ASTR in the ovaries (Supplementary Fig. 2c ), suggesting that the 3ʹ end of sisR-1 is required for target suppression. Furthermore, overexpression of sisR-1 caused an increase in the number of GSCs (appearance of germaria with four GSCs, Fig. 2f–h ), confirming that sisR-1 is sufficient to promote GSC–niche occupancy cell autonomously. However, no significant increase in GSCs was observed when we overexpressed sisR-1 containing mutations at the 3ʹ ends (Fig. 2h and Supplementary Fig. 2d, e ), indicating that the 3ʹ end is required for its function. We next examined the cellular mechanisms by which sisR-1 promotes GSC maintenance. Firstly, we did not observe any increase in cell death in sisR-1 RNAi GSCs (Supplementary Fig. 2f–h ), indicating that GSC loss was not due to apoptosis. GSCs are maintained by adhesion to the cap cells via E-Cadherin, and adhesion molecules are essential for niche occupancy during stem cell competition [30] , [31] , [32] , [33] , [34] . We observed that the expression of E-Cadherin between GSCs and cap cells was frequently low in sisR-1 RNAi ovaries (Fig. 2i–l , arrowheads ), suggesting that GSCs may be lost due to poor adhesion to the niche. Indeed, overexpression of E-Cadherin suppressed the GSC loss phenotype. (Fig. 2q and Supplementary Fig. 2k–n ). Egg chambers with overexpression of sisR-1 had higher levels of E-Cadherin compared to controls (Supplementary Fig. 2i, j ), indicating that sisR-1 regulates germline-soma cell adhesion. However, a previous report showed that overexpression of E-Cadherin alone is not sufficient to increase GSC number [35] , suggesting that sisR-1 regulates GSCs via cell adhesion and additional mechanisms. Overexpression of a Trim-NHL protein Mei-P26 in GSCs can lead to precocious differentiation [36] , [37] . Mei-P26 expression is low in GSCs and increases upon differentiation (Fig. 2m ) and therefore needs to be carefully regulated [37] , [38] . In sisR-1 RNAi ovaries, GSCs were frequently seen to upregulated Mei-P26, which was never seen in controls (Fig. 2m–p , arrowheads ). To investigate if GSC differentiation in sisR-1 RNAi ovaries was due to upregulation of Mei-P26, we remove a copy of mei-P26 . This experiment resulted in a suppression of the sisR-1 RNAi phenotype (Fig. 2q and Supplementary Fig. 2o, p ). In addition, we did not observe any defects on the decapentaplegic pathway and Bag-of-marbles expression (Supplementary Fig. 2q–ab ). Together, our data reveal that sisR-1 promotes GSC–niche occupancy via at least two genetic pathways: (1) promoting GSC–niche association via E-Cadherin and (2) repression of a differentiation factor Mei-P26. sisR-1 regulates GSC–niche occupancy via ASTR and rga In Drosophila , sisR-1 regulates rga via a negative feedback loop by repressing a cis-natural antisense transcript called ASTR (Fig. 3a ) [5] . It was shown previously that sisR-1 represses the abundance of ASTR , while ASTR functions as a positive regulator of rga expression. Therefore, ASTR functions as an intermediate between sisR-1 and rga in a negative feedback mechanism. Expression of rga and ASTR was detected during the early stages of oogenesis suggesting an active sisR-1 axis (Supplementary Fig. 3a–c ). Since sisR-1 represses ASTR , we expected that ASTR RNAi flies to mimic the phenotype of sisR-1 overexpression flies. As expected, knockdown of ASTR resulted in an increase in GSC–niche occupancy (Fig. 3b, j ). Overexpression of ASTR led to a significant change in distribution of germaria to having less GSCs (Supplementary Fig. 3d, e ), confirming that ASTR limits GSC–niche occupancy. Importantly, the GSC loss phenotype in sisR-1 RNAi was rescued by ASTR knockdown (Fig. 3c, d, j ), in agreement with the model that ASTR is downstream of sisR-1 in the regulation of GSC–niche occupancy. Since the ASTR RNAi phenotype was significantly altered by sisR-1 RNAi, it also suggests that sisR-1 may have additional targets or the ASTR RNAi was partial. Fig. 3 DIP1 regulates GSC–niche occupancy by repressing sisR-1 . a The sisR-1/ASTR/rga genetic pathway. b – i , k – m , o – q Confocal images of germaria of the indicated genotypes stained for alpha-Spectrin ( green ) and Vasa ( red ). Scale bar : 10 µM. Asterisks (*) mark the GSCs. j , n , r Charts showing the percentages of germaria with the indicated number of GSCs of the indicated genotypes. * P < 0.05, ** P < 0.01. Fisher’s exact test ( j , r ). Wilcoxon test ( n ). N = 20. Black asterisks are used when compared to control, red asterisks are used when compared to the respective RNAi or overexpression lines ( sisR-1 RNAi, ASTR RNAi. DIP1 RNAi and DIP1 OE). Red arrowhead in n indicates the appearance of germaria with four GSCs that are very rarely seen in controls. s A model for the regulation of GSC–niche occupancy by sisR-1 Full size image Next, we observed an increase in GSC–niche occupancy in rga RNAi flies (Fig. 3e, j and Supplementary Fig. 3f ). Reciprocally, overexpression of Rga resulted in a decrease in GSCs (Fig. 3f, j and Supplementary Fig. 3g ). Knockdown of rga suppressed the GSC loss phenotype in sisR-1 RNAi flies (Fig. 3g, h, j ). This result is consistent with the pathway that sisR-1 represses rga . Finally, overexpression of rga suppressed the ASTR RNAi phenotype (Fig. 3i, j ), placing rga downstream of ASTR . Taken together, our genetic analyses established a role for the sisR-1 axis in regulating GSC–niche occupancy in the Drosophila ovaries. DIP1 regulates GSC number by repressing sisR-1 Having found that sisR-1 regulates GSC self-renewal via ASTR and rga , we further investigated if DIP1 functions to regulate GSC–niche occupancy by modulating the levels of sisR-1 . Knockdown of DIP1 led to an increase in the percentage of germaria having  > 2 GSCs (Fig. 3k, n ). This result was confirmed in the DIP1 mutant, which also showed an increase in germaria having  > 2 GSCs (Supplementary Fig. 1d , arrowhead ). Furthermore, overexpression of DIP1 using MTD-Gal4 resulted in a significant decrease in GSCs (Fig. 3o, p, r ). To determine if DIP1 regulates GSCs through sisR-1 , we knocked down sisR-1 expression in DIP1 RNAi flies. In this situation, the GSC increase phenotype seen in DIP1 RNAi flies was indeed suppressed (Fig. 3l–n ). We further asked if overexpression of sisR-1 could suppress the DIP1 overexpression phenotype. In flies that overexpressed both sisR-1 and DIP1 under the control of MTD-Gal4 , the number of GSCs was reverted to wild-type level (Fig. 3q, r ). Together, our results put forward a model that DIP1 limits the steady-state levels of sisR-1 to maintain GSC homeostasis in the niche (Fig. 3s ). 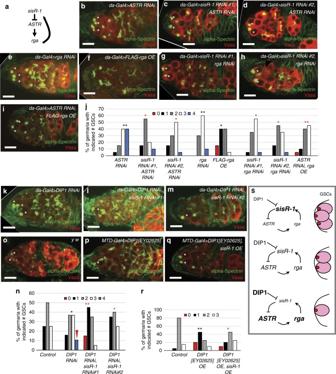Fig. 3 DIP1regulates GSC–niche occupancy by repressingsisR-1.aThesisR-1/ASTR/rgagenetic pathway.b–i,k–m,o–qConfocal images of germaria of the indicated genotypes stained for alpha-Spectrin (green) and Vasa (red).Scale bar: 10 µM.Asterisks(*) mark the GSCs.j,n,rCharts showing the percentages of germaria with the indicated number of GSCs of the indicated genotypes. *P< 0.05, **P< 0.01. Fisher’s exact test (j,r). Wilcoxon test (n).N= 20.Black asterisksare used when compared to control,red asterisksare used when compared to the respective RNAi or overexpression lines (sisR-1 RNAi, ASTRRNAi.DIP1RNAi andDIP1OE).Red arrowheadinnindicates the appearance of germaria with four GSCs that are very rarely seen in controls.sA model for the regulation of GSC–niche occupancy bysisR-1 A model for sisR-1 -mediated silencing Next, we attempted to gain some insights to the mechanism of sisR-1 -mediated ASTR silencing. We refer “3ʹ end” as the region of sisR-1 that overlaps with the 3ʹ end of ASTR by 76 nucleotides (nt) (Fig. 4a ), while “3ʹ tail” refers to the 29 nt region that binds to ASTR based on its predicted secondary structure (Fig. 4b ) [5] . We have shown that the 3ʹ tail of sisR-1 is necessary for silencing of ASTR (Supplementary Fig. 2a–c ). To test if the 3ʹ tail is sufficient for target degradation, we replaced the 3ʹ tail with an antisense element that base pairs with a nuclear long ncRNA rox2 (Supplementary Fig. 4a, b ). Ectopic expression of sisR-rox2 in S2 cells and in vivo did not lead to a significant downregulation of endogenous rox2 (Supplementary Fig. 4c, d ), indicating that the 3ʹ tail is not sufficient for target degradation. Taken together, our data suggest that the 3ʹ tail of sisR-1 is necessary but not sufficient for target repression. Fig. 4 A model for sisR-1 -mediated silencing of ASTR . a Drawing showing that sisR-1 and ASTR can form a 76 nt dsRNA at the 3ʹ ends. Not drawn to scale. b Drawing showing the targeting of ASTR by the 3ʹ tail (29 nt) in sisR-1 . c Drawing showing that sisR-rox1 and rox1 can form a 76 nt dsRNA at the 3ʹ ends. Not drawn to scale. d , e Predicted secondary structures of d wild-type sisR-1 and e chimeric sisR-rox1 . Orange : region of 76 nt that base pairs with rox1 . Red : compensatory mutations introduced to maintain the secondary structure. f RT-PCR showing the expression of sisR-rox1 transgene in male flies. g RT-qPCR showing the downregulation of rox1 ( black bars ) but not U85 ( white bars ) in control versus sisR-rox1 expressing male flies. N = 3–4 biological replicates. Student’s t -test was performed. Error bars represent s.d. h Northern blots (from at least two biological replicates) showing the relative abundance of ASTR between 2–14 h and 14–24 h embryos in y w control, dicer-2 L811fsX and ago 414 mutants. 18, 28S rRNA was used as loading controls. Numbers below indicate relative band intensities of ASTR normalized to rRNA quantified using ImageJ software. i A possible model of how sisR-1 may mediate decay of ASTR Full size image Next, we tested whether complementary base pairing between the 76 nt 3ʹ end of sisR-1 with the target is sufficient for target degradation. We replaced the 3ʹ end of sisR-1 with a 76 nt antisense element against an endogenous long ncRNA rox1 to design a chimeric sisR-1 (named sisR-rox1 ) (Fig. 4c–e ). Compensatory mutations were also introduced to the regions that base pair with the new 76 nt end sequences to preserve the secondary structure as much as possible (Fig. 4d, e , red : compensatory mutations, orange : 76 nt mutations). When ectopically expressed in the adult males (Fig. 4f ), sisR-rox1 could downregulate the expression of rox1 (Fig. 4g ). Although the fold-change in rox1 level was modest, it was statistically significant ( P value = 0.02). As endogenous expression of rox1 was high and comparable to housekeeping gene actin5C , a ~20% change was considerable in terms of copy number. Furthermore, the effect was specific to rox1 as another nuclear long ncRNA U85 remained unchanged in sisR-rox1 expressing flies (Fig. 4g ). Dicer-2 (Dcr-2) has been shown to localize to and function in the nucleus in Drosophila and human cells [39] , [40] , [41] , [42] . In vitro studies have shown that a ~40 nt duplex is sufficient for Dcr-2-mediated cleavage [43] . In wild types, endogenous ASTR is highly expressed in the early embryos (2–14 h) and dramatically downregulated in the late embryos (14–24 h) (Fig. 4h ) [5] . In dcr-2 mutants, the downregulation of ASTR is severely perturbed in late embryos (Fig. 4h ), consistent with a requirement for Dcr-2 (Fig. 4h ). Since Dcr-2 is a component of the endogenous siRNA pathway, we asked if the downstream effector Argonaute2 (Ago2) is also required for ASTR silencing. In ago2 mutants, we did not observe any defects in the downregulation of ASTR in the late embryos (Fig. 4h ), further suggesting that siRNAs are not involved. This observation is very similar to what was reported in human and mice where Dicer1 regulates Alu RNA independent of its RNA interference function [40] . Our results are consistent with a model in which a naturally occurring sisRNA sisR-1 represses its target via two sequential steps: (1) target recognition via complementary base pairing of 3ʹ tail to its target, and (2) more extensive dsRNA formation between sisR-1 and its target, which is cleaved by endonuclease Dcr-2 (Fig. 4i ). DIP1 localizes as foci in the nuclei of the germline cells Many proteins that are involved in RNA metabolism localize to specific nuclear or cytoplasmic bodies such as Cajal bodies, Histone Locus Bodies (HLBs), Processing bodies, nuage, and Yb bodies [44] , [45] , [46] , [47] , [48] , [49] . To investigate the cellular localization of DIP1, we performed immunostaining using our DIP1 antibody. DIP1 localizes as nuclear foci in germline cells in the germaria (Supplementary Fig. 1e ), similar to what was previously reported [23] . The staining was dramatically reduced in DIP1 mutant ovaries (Supplementary Fig. 1f ). In the transcriptionally active nurse cells in the stage 5 egg chamber, DIP1 also localizes as discrete nuclear foci (Supplementary Fig. 1g, h ). However, DIP1 does not form nuclear foci in the transcriptionally quiescent oocyte nucleus and cyst cells during mitosis (Supplementary Fig. 1i, j ), suggesting that formation or maintenance of DIP1 nuclear foci may be associated with active transcription. In the testes, DIP1 also forms nuclear foci in the primary spermatocytes. Discrete nuclear foci could be seen during the transition from spermatogonia to primary spermatocytes (Supplementary Fig. 1k, l ). When the primary spermatocytes grow larger with massive transcription of fertility genes, DIP1 staining filled the entire nuclei (Supplementary Fig. 1m ). Furthermore, DIP1 staining was not detected in the sperm bundles where no transcription occurs (Supplementary Fig. 1n ). Taken together, our data indicated that DIP1 localizes as nuclear foci in transcriptionally active germline cells. We further generated HA-tagged DIP1 transgenic flies (Supplementary Fig. 1o, p ). When expressed in germline cells, HA-DIP1 exhibited the same nuclear foci that were detected by DIP1 antibody (Supplementary Fig. 1q, r ). To test if RNA is required for the maintenance of DIP1 nuclear foci, we treated ovaries with RNase A. Indeed, after treatment with RNase A, HA-DIP1 nuclear foci became diffused compared to mock treated control ovaries (Supplementary Fig. 1s, t ). 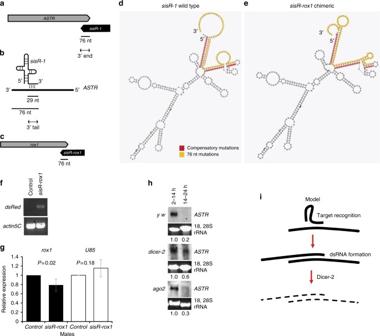Fig. 4 A model forsisR-1-mediated silencing ofASTR.aDrawing showing thatsisR-1andASTRcan form a 76 nt dsRNA at the 3ʹ ends. Not drawn to scale.bDrawing showing the targeting ofASTRby the 3ʹ tail (29 nt) insisR-1.cDrawing showing thatsisR-rox1androx1can form a 76 nt dsRNA at the 3ʹ ends. Not drawn to scale.d,ePredicted secondary structures ofdwild-typesisR-1andechimericsisR-rox1.Orange: region of 76 nt that base pairs withrox1.Red: compensatory mutations introduced to maintain the secondary structure.fRT-PCR showing the expression ofsisR-rox1transgene in male flies.gRT-qPCR showing the downregulation ofrox1(black bars) but notU85(white bars) in control versussisR-rox1expressing male flies.N= 3–4 biological replicates. Student’st-test was performed.Error barsrepresent s.d.hNorthern blots (from at least two biological replicates) showing the relative abundance ofASTRbetween 2–14 h and 14–24 h embryos iny wcontrol,dicer-2L811fsXandago414mutants. 18, 28S rRNA was used as loading controls. Numbers below indicate relative band intensities ofASTRnormalized to rRNA quantified using ImageJ software.iA possible model of howsisR-1may mediate decay ofASTR These data are consistent with the idea that maintenance of DIP1 foci may require the transcripts that are present in the nucleus. Satellite bodies decorate the fourth chromosomes We characterized the DIP1 nuclear foci more carefully by examining the huge nurse cells of the later stage egg chambers, which allow better resolution of the nuclear localization. In stage 7/8 nurse cells, when the chromosomes become polyploid, DIP1 localizes as discrete round bodies around a DAPI dense region (Fig. 5a , arrowhead ). This DAPI dense region was previously shown to be the heterochromatin of the fourth chromosomes and each nurse cell contains only one such region because homologous chromosomes are paired and clustered during this stage of oogenesis [50] . Staining with a marker for the fourth chromosome Paint of fourth (POF) confirmed that this DAPI dense region is the chromosome four (Fig. 5b , arrowhead ) [51] . HA-DIP1 also localized as bodies that decorated the fourth chromosomes (Fig. 5c , arrowheads ). In general, the staining pattern of DIP1 differs from that of POF. While POF localizes on the chromosomes, DIP1 appears as small foci that surround or decorate the chromosomes. We named these DIP1 defined bodies satellite bodies because they resemble satellites that revolve around the planet (DAPI-dense dot). Fig. 5 Satellite bodies are DIP1-positive nuclear bodies that decorate the fourth chromosomes. a A stage 7/8 nurse cell stained for DIP1 and DAPI. b , d , e A stage 7/8 nurse cell stained for b POF, d Coilin, and e LSM10. c A stage 7/8 egg chamber expressing HA-DIP1 protein under MTD-Gal4 , stained with anti-HA. f Two stage 10/11 nurse cells stained for DIP1 and DAPI. g A magnified view of satellite bodies in f . h A stage 10/11 nurse cell stained for POF and DAPI. Arrowheads point to DAPI-dense regions of fourth chromosomes. i , j Follicle cells stained for i DIP1 and j POF. k , l S2 cells stained for k DIP1 and l POF. White arrowheads point to chromosome four associated bodies, while yellow arrowheads point to bodies that do not associate with chromosome four. Scale bar : 10 µm Full size image Satellite bodies appear to define a novel class of nuclear bodies as other known nuclear bodies such as Cajal body and HLB do not associate with chromosome four (Fig. 5d, e , arrowheads ) [44] . When the chromosomes become polytenized in the stage 10/11 nurse cells, satellite bodies become elongated in shape. Nevertheless, they still associate with the fourth chromosome as evident by the presence of POF staining around the DAPI-dense region (Fig. 5f–h , arrowheads ). Cytoplasmic bodies such as the nuage and balbiani bodies are only present in germline cells [48] . Besides germline cells, satellite bodies are also present in the somatic follicle cells. The fourth chromosomes are almost always associated with a DIP1-positive satellite body (Fig. 5i , white arrowheads ). In some cells, there are also additional DIP1-positive bodies that are not associated with chromosome four (Fig. 5i , yellow arrowheads ). The genomic association of these bodies is currently unclear and requires further investigation. This localization pattern is different from that of POF, which only labeled the fourth chromosomes (Fig. 5j , arrowheads ). Similar bodies that associate and do not associate with the fourth chromosomes were also found in cultured S2 cells (Fig. 5k, l ). DIP1 suppresses the abundance of INE-1 sisRNAs Since the localizations of the nucleolus and HLB correlate with a high concentration of transcription of specific RNA species, we asked whether the fourth chromosome could be a rich source of a specific class of RNA molecules. The Drosophila chromosome four is a very small chromosome and contains a very high density of the INE-1 transposable element sequences (Fig. 6a and Supplementary Fig. 5 ) [52] , [53] , [54] . It is also rich in essential genes and is transcriptionally active. Majority of the INE-1 elements are present in the introns of the genes, in either single or multiple copies, and are present in both orientations (Fig. 6b and Supplementary Fig. 5 ) [53] . Since intronic INE-1 sequences are co-transcribed with the host genes, chromosome four may be a rich source of INE-1 sisRNAs. Fig. 6 DIP1 suppresses the level of INE-1 sisRNAs. a Chart showing the number of INE-1 insertions per Mbp of DNA on the different chromosomes in Drosophila melanogaster . b Genetic loci for eyeless ( ey ) and CamKII showing the location of INE-1 insertions in the introns. Red bars indicate the gene-specific INE-1 sisRNAs amplified in c . c RT-PCR showing the presence of ey , CamKII and INE-1 sisRNAs in unfertilized eggs. gDNA, genomic DNA. d Strand-specific RT-PCR showing the presence of both anti-sense and sense ey sisRNAs in unfertilized eggs. e Confocal images showing the localization of INE-1 sisRNAs ( Green ) and DAPI ( Red ) in a nurse cell nucleus. Arrowheads point to DAPI-dense regions of fourth chromosomes. f Confocal images showing the localization of INE-1 sisRNAs ( Green ), DIP1 ( Red ), and DAPI ( Blue ) in a nurse cell nucleus. Arrowheads point to DAPI-dense regions of fourth chromosomes. g RT-qPCR showing the relative levels of INE-1, HeT-A , CG32000 , and CG2316 in control and DIP1 mutant ovaries. h RT-qPCR showing the relative levels of INE-1, ey and CamKII in MTD-Gal4 control and MTD-Gal4 > HA-DIP1 ovaries. * P < 0.01. Two-tailed t -test. N = 3 independent biological replicates. Error bars represent s.d. i Working model on the role of DIP1-positive satellite bodies in regulating the abundance of INE-1 sisRNAs in Drosophila Full size image Indeed, INE-1 containing intronic transcripts are processed into sisRNAs in unfertilized eggs, which store a pool of stable and mature RNAs without any contamination from nascent transcripts. We detected the presence of INE-1 sisRNAs in unfertilized eggs via RT-PCR using generic primers for INE-1 sequences and intron-specific primers for two chromosome four genes eyeless ( ey ) and CamKII (Fig. 6b, c ). The CamKII sisRNA was also previously detected in eggs to be ~10% the level of its parent gene [5] . Interestingly, both strands of the INE-1 sisRNAs from the ey gene were present in the eggs (Fig. 6d ), implying that they may form dsRNAs. Fluorescent in situ hybridization showed that INE-1 sisRNAs clustered around and on the fourth chromosomes, although they were also present, to a lesser extent, in other regions of the nucleus (Fig. 6e ). 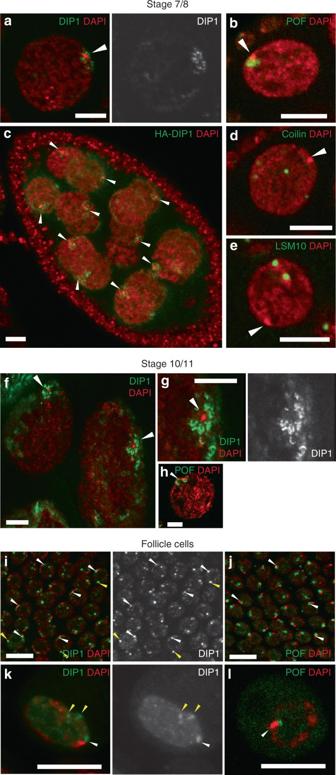Fig. 5 Satellite bodies are DIP1-positive nuclear bodies that decorate the fourth chromosomes.aA stage 7/8 nurse cell stained for DIP1 and DAPI.b,d,eA stage 7/8 nurse cell stained forbPOF,dCoilin, andeLSM10.cA stage 7/8 egg chamber expressing HA-DIP1 protein underMTD-Gal4, stained with anti-HA.fTwo stage 10/11 nurse cells stained for DIP1 and DAPI.gA magnified view of satellite bodies inf.hA stage 10/11 nurse cell stained for POF and DAPI.Arrowheadspoint to DAPI-dense regions of fourth chromosomes.i,jFollicle cells stained foriDIP1 andjPOF.k,lS2 cells stained forkDIP1 andlPOF.White arrowheadspoint to chromosome four associated bodies, whileyellow arrowheadspoint to bodies that do not associate with chromosome four.Scale bar: 10 µm 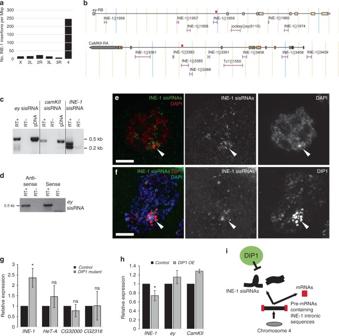Fig. 6 DIP1 suppresses the level of INE-1 sisRNAs.aChart showing the number of INE-1 insertions per Mbp of DNA on the different chromosomes inDrosophila melanogaster.bGenetic loci foreyeless(ey) andCamKIIshowing the location of INE-1 insertions in the introns.Red barsindicate the gene-specific INE-1 sisRNAs amplified inc.cRT-PCR showing the presence ofey,CamKIIand INE-1 sisRNAs in unfertilized eggs. gDNA, genomic DNA.dStrand-specific RT-PCR showing the presence of both anti-sense and senseeysisRNAs in unfertilized eggs.eConfocal images showing the localization of INE-1 sisRNAs (Green) and DAPI (Red) in a nurse cell nucleus.Arrowheadspoint to DAPI-dense regions of fourth chromosomes.fConfocal images showing the localization of INE-1 sisRNAs (Green), DIP1 (Red), and DAPI (Blue) in a nurse cell nucleus.Arrowheadspoint to DAPI-dense regions of fourth chromosomes.gRT-qPCR showing the relative levels of INE-1,HeT-A,CG32000, andCG2316in control andDIP1mutant ovaries.hRT-qPCR showing the relative levels of INE-1,eyandCamKIIinMTD-Gal4control andMTD-Gal4 > HA-DIP1ovaries. *P< 0.01. Two-tailedt-test.N= 3 independent biological replicates.Error barsrepresent s.d.iWorking model on the role of DIP1-positive satellite bodies in regulating the abundance of INE-1 sisRNAs inDrosophila These INE-1 sisRNAs are closely associated with the DIP1-positive satellite bodies (some co-localize with DIP1, while others in close proximity to DIP1), suggesting some regulatory relationships (Fig. 6f ). Furthermore, we also detected interaction between DIP1 and INE-1 sisRNAs in S2 cells (Fig. 1c ). Since DIP1 represses sisR-1 , we examined if DIP1 also regulates INE-1 sisRNA abundance. In DIP1 mutant ovaries, the steady-state abundance of INE-1 sisRNAs was upregulated, suggesting that DIP1 represses INE-1 sisRNAs (Fig. 6g ). We did not observed a significant change in the expression of HeT-A (a telomeric retrotransposon regulated by the piRNA pathway) (Fig. 6g ) [48] , suggesting that DIP1 is not a component of the piRNA pathway. We also did not observed any changes in the expression of two other chromosome four genes ( CG32000 and CG2316 ) that have INE-1 sequences in their introns (Fig. 6g ), suggesting that DIP1 does not regulate the transcriptional state of the fourth chromosomes in general. Furthermore, overexpression of DIP1 in the germline cells led to a decrease in the level of INE-1 sisRNAs, but not for parental genes such as ey and CamKII (Fig. 6h ), confirming a role of DIP1 in repressing INE-1 sisRNAs. Together, our data reveal the identification of DIP1 as a repressor of sisR-1 and INE-1 sisRNAs at the post transcriptional level (Fig. 6i ). Although DIP1 seems to regulate INE-1 sisRNAs in the satellite bodies, the regulation of sisR-1 , which is not on the fourth chromosome, by DIP1 presumably occurs outside the satellite bodies. Our results reveal the importance of the regulation of sisRNA activity/expression in GSC–niche occupancy. We propose that the sisR-1 axis maintains GSCs in the niche, however, uncontrolled accumulation of sisR-1 due to its unusual stability can lead to increase number of GSCs at the niche. DIP1 in turn limits the build-up of sisR-1 to maintain ~2 GSCs per niche (Fig. 3s ). GSC–niche occupancy is highly regulated by homeostatic mechanisms via negative feedback loops at the cellular and molecular levels [33] , [55] , [56] . Mis regulation of the niche may pose a problem as it allows for a greater chance of GSCs to accumulate mutations that may lead to tumor formation [31] , [56] , [57] . On the other hand, mechanisms that promote GSC–niche occupancy may be important to facilitate the replenishment of GSCs during aging [34] , [58] , [59] . Understanding the control of stem cell-niche occupancy will provide important insights to reproduction, cancer, and regenerative medicine. In a large-scale RNAi screen for genes that regulate GSC self-renewal and differentiation, rga was identified as a gene required for GSC differentiation [29] . How rga regulates GSC self-renewal is currently unknown but our data suggest that GSC–niche adhesion and Mei-P26 are involved. The rga gene encodes for the NOT2 protein in the CCR4 deadenylase complex [60] , [61] , [62] . Surprisingly, studies have shown that other components of the CCR4 complex such as CCR4, Not1, and Not3 function in promoting GSC maintenance [35] , [36] . Interestingly, Twin has been proposed to function with distinct partners to mediate different effects on GSC fates [35] . This suggests that other components such as CCR4 can also have additional functions outside the CCR4–NOT deadenylase complex in mediating GSC maintenance, thus affecting GSCs in opposite ways to Rga. Here, we put forward a proposed model for sisR-1 -mediated silencing. We hypothesize that folded sisR-1 harboring a 3ʹ tail may form a ribonucleoprotein complex, which confers its stability, and allows scanning for its target via its 3ʹ tail. Binding of the 3ʹ tail to the target may promote local unwinding of sisR-1 as the 3ʹ end of ASTR invades to form a more stable 76 nt duplex. We show that, in principle, it is possible to design a chimeric sisRNA to target a long ncRNA of interest such as rox1 . In future, sisRNA can be potentially developed as tools to regulate nuclear RNAs of interest. Clearly, the efficiency and specificity of sisRNA-mediated silencing need to be optimized. Because sisRNA-mediated target degradation requires a more extensive base-pairing between sisRNA and the target, the chances of off-target effects ought to be lower than siRNAs and antisense oligonucleotides. In broader terms, our study provides a paradigm, which encourages exploration of whether other sisRNAs or ncRNAs utilize a similar silencing strategy as sisR-1 . We describe a nuclear body (named satellite body) that associates with the fourth chromosomes. Satellite body adds to an existing group of nuclear bodies (nucleolus, HLB, and pearl) that associate with specific genomic loci [63] . It is generally believed that formation of such nuclear bodies correlates with a high concentration of RNA transcribed from the tandemly repeated gene loci. The formation of satellite bodies around the fourth chromosomes probably reflects a high concentration of DIP1 in regulating INE-1 sisRNAs transcribed there. The formation of satellite bodies may be promoted by the high concentration of INE-1 sisRNAs transcribed on the fourth chromosomes, and may facilitate the decay of INE-1 sisRNAs (Fig. 6i ). We speculate that in the nucleoplasm, DIP1 that does not form observable satellite bodies is sufficient to regulate sisRNAs such as sisR-1 transcribed from other chromosomes. Since DIP1 is a dsRNA binding protein, it may bind to mature sisRNAs to destabilize them. It may do so by recruiting RNA degradation factors (such as nuclear exosomes) or introducing RNA modification to “mark” sisRNAs for degradation. In future, it will be important to identify more components of the satellite bodies and their dynamics during differentiation and in response to stimuli in order to better understand the molecular mechanism of sisRNA metabolism. Fly strains The following fly strains were used in this study: y w , MTD-Gal4 [64] , da-Gal4, sisR-1 RNAi-1/CyO [5] , sisR-1 RNAi-2/CyO [5] , ASTR RNAi/TM3 [5] , UAS-sisR-1 [5] , rga RNAi GL00386 (Bloomington #35460), DIP1 EY02625 (Bloomington #15577), DIP1 RNAi GL00242 (Bloomington #35333), dad-GFP (enhancer trap), P[bam]-GFP, mei-P26 mfs1 (Bloomington #25919), UASp-shg (Bloomington #58494), dicer-2 L811fsX 16 and ago 414 [65] . Before dissection, females were fed with wet yeast for 7 days (7-day old) at 25 °C. Note that it has been verified previously that sisR-1 RNAi knocked down sisR-1 but not the parental rga mRNA [5] . Locations of RNAi constructs were indicated in Fig. 1c . For generation of sisR-1 overexpression clones, hsFLP;nos>STOP>Gal4,UAS-GFP flies [66] were crossed to UAS-sisR-1 flies. Flies were heat shocked at 37 °C two times daily at 7–8 h intervals for three consecutive days and dissected for staining one day after the last heat shock. In the overexpression assays, da-Gal4 was used when combined with UASp transgenes, while MTD-Gal4 was used when combined with UASt transgenes, to achieve maximum overexpression efficiencies. Generation of transgenic flies PCR of rga full-length coding sequence (CDS) was performed using primers, CACC- rga FW (5′ CACCATGGCGAATTTAAATTTTCAACAACCC 3′) and rga Rv (5′ TTATACAGACTGTCCATTCATAAACGCACTTATATTGG 3′). PCR of ASTR full-length sequence was performed using primers, CACC- ASTR FW (5′ CACCCAAAGTTAATCAGATATTCGGGTGG 3′) and ASTR Rv (5′ TGCAATCTCATTTACTTTGAAACATGAT 3′). For UASp-HA-DIP1-c transgenic flies primers used were cacc-DIP1-c Fw CACCATGAAGCGAAATCGTCGTGC and DIP1-c Rv AGTGGTGTCGCTGTAGGTGA. Transgenic flies expressing DIP-1-c-HA were not generated because C-terminal tagged DIP1 protein was not stable when expressed in S2 cells. The PCR products were purified, cloned into pENTR TOPO vector (Invitrogen) and transformed into One Shot chemically competent Escherichia coli cells. Plasmids were checked by sequencing. LR reactions were then carried out using Gateway LR Clonase II Enzyme mix (Invitrogen). Transgenic flies were generated by BestGene using P-element-mediated insertion [67] . Transgenic flies expressing dsRed-sisR-1-myc was generated as previously described [5] . Intronic fragments were chemically synthesized and sub-cloned into linearized UASt-dsRed-myc plasmid. Injection was done by BestGene Inc. DIP1 antibody Two independent affinity-purified polyclonal antibodies against full-length DIP1-c were generated in rabbits by GenScript. Both antibodies gave identical staining patterns. Immunostaining Immunostaining was performed as described previously [68] . Ovaries were fixed in a solution of 16% paraformaldehyde and Grace’s medium at a ratio of 2:1 for 10–20 min, rinsed and washed with PBX solution (phosphate-buffered saline containing 0.2% Triton X-100) three times for 10 min each, and pre-absorbed for 30 min in PBX containing 5% normal goat serum. Ovaries were incubated overnight with primary antibodies at room temperature, washed three times for 20 min each with PBX before a 4 h incubation with secondary antibodies at room temperature. Ovaries were again washed three times for 20 min each with PBX. Primary antibodies used in this study are as follows: mouse monoclonal anti-α-Spectrin (3A9, 1:1; Developmental Studies Hybridoma Bank), rabbit anti-Rga (1:500, kind gift from Claudia Temme and Elmar Wahle) [61] , guinea pig anti-Vasa (1:1000, kind gift from Toshie Kai), rabbit anti-pMad (1:50; Cell Signaling Technology #9516), mouse anti-Bam (1:10, Developmental Studies Hybridoma Bank), mouse anti-GFP (3E6, 1:500, Invitrogen #A11120), rat anti-E-Cadherin (1:200, Developmental Studies Hybridoma Bank), rabbit anti-Mei-P26 (1:1000, kind gift from Paul Lasko) [38] , rabbit anti-DIP1 (1:100, this study), rabbit anti-Coilin (1:2,000, kind gift from Joseph Gall), rabbit anti-LSM10 (1:2,000, kind gift from Joseph Gall), rabbit anti-POF (1:1,000, kind gift from Jan Larsson) and rat anti-HA (3F10, 1:500, Sigma #11867423001). Labeling of apoptotic cells were done using the TUNEL assay (Molecular Probes) in accordance to the manufacturer’s protocol. Images were taken with a Carl Zeiss LSM 5 Exciter Upright microscope and processed using Adobe Photoshop. RNA FISH RNA FISH was performed according to a published protocol [69] . DIG-labeled DNA probes for INE-1 were generated by PCR as described previously [5] . Ovaries were dissected in Grace’s medium, fixed for 20 min in PBTT with 4% formaldehyde. Ovaries were then rinsed and washed with PBT and followed by 10 min incubation in cold 80% acetone at −20 °C. The ovaries were washed and post-fixed for 10 min in PBT with 4% formaldehyde, followed by washing with PBT, rinsing in 1:1 PBT/hybridization solution, hybridization solution, and blocking in hybridization solution for at least 2 h at 42 °C. The samples were then incubated in the probe/hybridization mixture at 42 °C overnight. Next day, samples were washed with 3:1, 1:1, 1:3 hybridization solution/PBT and PBT at 42 °C, and then blocked and incubated in primary antibodies (anti-DIP-POD and rabbit anti-DIP1) for 2 h at room temperature. The samples were washed and Tyramide Signal Amplification was performed in accordance to the manufacturer’s protocol. Actinomycin D treatment Actinomycin D treatment was performed as previously described [5] . Ovaries were incubated in Grace’s medium containing 20 µg ml −1 actinomycin D with constant rocking at room temperature. RNase A treatment of ovaries Ovaries were dissected in Grace’s media at room temperature. Ovaries were incubated in Grace’s media containing either no chemicals (mock) or RNase A (100 µg ml −1 ) with rocking for 30 min at room temperature as described previously [5] . RNA extraction Tissues were homogenized in 1.5 ml Eppendorf tubes using a plastic pestle and RNA was extracted using the TRIzol extraction protocol (Ambion) or the Direct-zol RNA miniprep kit (Zymo Research). RNA was quantified using a Nanodrop spectrophotometer to ensure equivalent loading for subsequent experiments. RNA immunoprecipitation S2 cells that survive in serum-free medium were obtained from Steve Cohen’s laboratory. Immunoprecipitation was performed as described with minor modifications [70] . Cells were lysed in protein extraction buffer (50 mM Tris-HCl pH 7.5, 150 mM NaCl, 5 mM MgCl 2 , 0.1% NP-40) supplemented with Protease Inhibitor Cocktail (Roche). Lysates were then pre-cleared with protein A/G agarose beads (Merck Millipore). Three microlitre of rabbit anti-DIP1 was added and incubated for 3 h at 4 °C. Protein A/G agarose beads were then added and incubated for another 1 h. After incubation, beads were washed three times with protein extraction buffer, and RNA was extracted using the Direct-zol RNA miniprep kit (Zymo Research). RT-PCR RT-PCR was performed as previously described [5] . For standard RT-PCR, total RNA was reverse transcribed with random hexamers for 1 h using AMV-RT (New England Biolabs), M-MLV RT (Promega) or Superscript III (Invitrogen). Strand-specific RT-PCR was performed using SuperScript III RT (Invitrogen) or M-MLV RT (Promega). PCR was carried out using the resulting cDNA. For quantitative PCR (qPCR), SYBR Fast qPCR kit master mix (2×) universal (Kapa Biosystems, USA) was used with addition of ROX reference dye high and carried out on the Applied Biosystems 7900HT Fast Real-Time PCR system. Oligo sequences were reported previously [5] . DIP1 Fw: 5′ TAATACGACTCACTATAGGGAGAAAGAAGTTGCGACAGAACCG 3′ and DIP1 Rv: 5′ TAATACGACTCACTATAGGGAGACGAACAGCTTGTAGATGGCA 3′. CamKII INE-1 Fw TGGGCTATTTTTAGGCGTCA, CamKII INE-1 Rv TATGAACGCGTCGATCTCAG, ey INE-1 Fw CGGAAAATGCCAAGGACTAA, ey INE-1 Rv GCTAAATGGGCACACTCGTC, INE-1 Fw GGCCATGTCCGTCTGTCC, INE-1 Rv AGCTAGTGTGAATGCGAACG, rox1 forward TGCAGTGGCAGTTTCTTCTG, rox1 reverse GGTCCGTGCAAAGCAGTAAT, rox2 forward TCTCCGAAGCAAAATCAAGC, rox2 reverse TGTTGCGTTCCAAGACACAT. Western blot Ovaries were dissected in Grace’s medium and homogenized in 2× sample buffer. Western blotting was performed as previously described [68] . Antibodies used were rabbit anti-Rga [61] (1:5000), mouse anti-FLAG M2 (1:5000, Sigma #F3165), mouse anti-Alpha Tubulin (clone DM1A, 1:10,000, Millipore #05-829), and rat anti-HA (3F10, 1:5,000, Sigma #11867423001). All uncropped western blots can be found in Supplementary Fig. 6 . Northern blotting Northern blotting was performed as described previously [5] . DIG-labeled DNA probes were made by PCR using genomic DNA as the template. To detect sisR-1 , RNA was run on an 8% polyacrylamide gel (8 M urea, 1× TBE buffer), and transferred onto a nylon membrane by electrophoresis. To detect, ASTR , RNA was run on a 0.8% agarose/formaldehyde gel and transferred onto a nylon membrane by capillary action. RNA was UV crosslinked to the membrane, pre-hybridized in salmon sperm DNA, and hybridized with probes in DIG Easy Hyb Granules (Roche) at 42 °C overnight. Next day, the membranes were washed once with 2× SSC and 0.1% SDS, and twice with 0.1× SSC and 0.1% SDS, followed by detection with the CDP-Star chemiluminescent substrate (Roche). Bioinformatics Annotation information of INE-1 all insertions and gene introns are from FlyBase. Bedtools intersect was used to extract INE-1 insertions located at introns. Custom scripts were used to convert the raw annotation data to bed format to upload into UCSC GB as custom tracks. The images were downloaded from custom tracks from UCSC GB. The custom tracks represent the INE-1 all insertions in the dm3 genome or insertions only in annotated introns. Statistical analysis At least 20 germaria from a total of 3–4 flies (6–8 ovaries) were sampled for each genotype. Fisher’s exact test was performed for all GSC counts except for Fig. 3n where Wilcoxon test was performed. No randomization or blinding was performed. Data availability The authors declare that all data supporting the findings of this study are available within the article and its supplementary information files or from the corresponding author upon reasonable request.